A long Stokes shift red fluorescent Ca2+indicator protein for two-photon and ratiometric imaging The introduction of calcium ion (Ca 2+ ) indicators based on red fluorescent proteins (RFPs) has created new opportunities for multicolour visualization of intracellular Ca 2+ dynamics. However, one drawback of these indicators is that they have optimal two-photon excitation outside the near-infrared window (650–1,000 nm) where tissue is most transparent to light. To address this shortcoming, we developed a long Stokes shift RFP-based Ca 2+ indicator, REX-GECO1, with optimal two-photon excitation at <1,000 nm. REX-GECO1 fluoresces at 585 nm when excited at 480 nm or 910 nm by a one- or two-photon process, respectively. We demonstrate that REX-GECO1 can be used as either a ratiometric or intensiometric Ca 2+ indicator in organotypic hippocampal slice cultures (one- and two-photon) and the visual system of albino tadpoles (two-photon). Furthermore, we demonstrate single excitation wavelength two-colour Ca 2+ and glutamate imaging in organotypic cultures. The development of genetically encoded Ca 2+ indicators has proven to be a great benefit to cell biology, as these tools have enabled the robust visualization and quantification of this key cytosolic second messenger in a diverse array of cell types and tissues [1] , [2] . The two most important classes of genetically encoded Ca 2+ indicators are the Förster resonance energy transfer-type (that is, cameleon) [3] , and the GCaMP-type [4] , [5] . GCaMP-type indicators are composed of the calmodulin (CaM) Ca 2+ binding protein and the CaM-binding region of chicken myosin light chain kinase (M13), fused to the C and N termini of a circularly permuted (cp) fluorescent protein (FP). The prototypical mechanism for a GCaMP-type indicator involves the Ca 2+ -dependent association of CaM and M13, causing a modification of the environment of the tyrosine-derived chromophore such that the fluorescent brightness or hue is modulated. Most typically, this modulation is attributable to changes in the effective p K a of the chromophore and concomitant changes in the relative populations of the protonated phenol and deprotonated phenolate forms [6] . Among the various GCaMP-type indicators reported in recent years are green fluorescent variants highly optimized for in vivo neuronal imaging [7] , photoconvertible variants [8] , and various new colours, including blue, cyan, yellow and red [9] , [10] , [11] , [12] . Of these new colours, red fluorescent indicators have the greatest potential to challenge the latest generation of highly optimized GCaMP variants [7] as the preferred tools for in vivo imaging. The versatility of currently available red FP-based Ca 2+ indicators has been demonstrated in various tissues and organisms including the retinotectal system in zebrafish [13] , mushroom body neurons in Drosophila [14] , [15] and chicken spinal cord [16] . Relative to more blue-shifted fluorophores, red fluorophores have the intrinsic advantages of improved tissue penetration for both the excitation and emission light, and lower autofluorescence and phototoxicity due to longer wavelength excitation. These favourable trends continue for wavelengths extending into the near-infrared (NIR) optical window ( ∼ 650–1,000 nm), where light penetrates the furthest into mammalian tissue due to minimal absorption by haemoglobin and water [17] , [18] . Despite substantial efforts to push RFPs [19] and RFP-based Ca 2+ indicators [10] to ever-longer excitation and emission wavelengths, even the most red-shifted fluorophores of the RFPs have negligible one-photon absorbance at wavelengths of 650 nm or above. An alternative approach to excite visible fluorophores is two-photon excitation [20] at NIR wavelengths that are approximately double (half the energy) the one-photon excitation maximum. However, as RFPs tend to have one-photon excitation peaks at 580–600 nm, their two-photon cross-section maxima typically lie beyond 1,000 nm [21] . At these wavelengths, absorption by water can lead to undesirable tissue heating, and, importantly, these wavelengths are out of tuning range of many commercial Ti-sapphire lasers. One effective solution to this problem is to exploit long Stokes shift RFPs, such as mKeima [22] , which have one-photon excitation maxima at wavelengths <500 nm and optimal two-photon cross-section at <1,000 nm. The ground state chromophore of a long Stokes shift RFP primarily exists in the protonated form. Typically, a proximal acidic group (that is, the carboxylate side chain of Asp or Glu) acts to destabilize the anionic phenolate form (absorbance ∼ 580 nm; fluorescence ∼ 600 nm) and stabilize the neutral phenol form (absorbance ∼ 460 nm; typically non-fluorescent). Illumination leads to formation of the excited state of the phenol form, which is associated with a decreased p K a . Excited state proton transfer (ESPT) occurs and the proton is transferred from the phenol moiety to the proximal acidic group, producing the phenolate form of the chromophore that emits its characteristic red fluorescence [23] . It has been reported that ESPT (and long Stokes shift spectral characteristics) can be engineered into RFPs, such as mKate, by introducing an acidic Glu or Asp residue at position 160, which is in close proximity to the phenol group of the chromophore [24] . Inspired by the X-ray crystal structure of the red fluorescent Ca 2+ indicator R-GECO1 (PDB ID 4I2Y) [9] , we reasoned that we could engineer it to undergo Ca 2+ -dependent ESPT. We expected that this would produce a long Stokes shift red fluorescent Ca 2+ indicator with a two-photon excitation maximum in the NIR window. Here, we describe our successful effort to develop, characterize and validate a genetically encoded long Stokes shift red fluorescent Ca 2+ indicator. Initial engineering of REX-GECO0.1 Our design for engineering a ratiometric red Ca 2+ indicator was inspired by reports of engineered monomeric RFPs with large Stokes shift [23] , [24] . Inspection of the X-ray crystal structure of R-GECO1 (PDB ID 4I2Y) [9] ( Fig. 1a ) revealed three residues (Ser64, Lys80 and Ile116; GCaMP numbering as in the PDB file 3EVR [6] ; Supplementary Fig. 1 ) that were near the phenolate moiety of the chromophore of R-GECO1 in the Ca 2+ -bound state. We reasoned that each of these residues could potentially serve to stabilize the phenol form and act as an excited state proton acceptor if mutated to an acidic residue. Lys80 was the most promising position owing to its direct electrostatic interaction with the phenolate moiety. To test our hypothesis, we created a genetic library in which the codons for Ser64, Lys80 and Ile116 were simultaneously randomized using a codon subset that encoded for a total of 624 different variants. This library was expressed in the pTorPE periplasmic expression vector [11] and thoroughly screened in a colony-imaging format by looking for clones that exhibited long Stokes shift red fluorescence (excitation at 438/24 nm and emission 609/57 nm). This screening led to the identification of an excitation ratiometric variant, designated as REX-GECO0.1, which harboured the Lys80Glu mutation. REX-GECO0.1 exhibits an excitation peak at ∼ 575 nm (that is, the phenolate form) in the Ca 2+ -free state and, on binding to Ca 2+ , this peak diminishes and a long Stokes shift excitation peak arises at ∼ 480 nm (that is, the phenol form). The excitation ratio ( R =red intensity with excitation at 450 nm divided by the red intensity with excitation at 580 nm) increases 6.5-fold ( R +Ca / R − Ca –1) on binding to Ca 2+ . 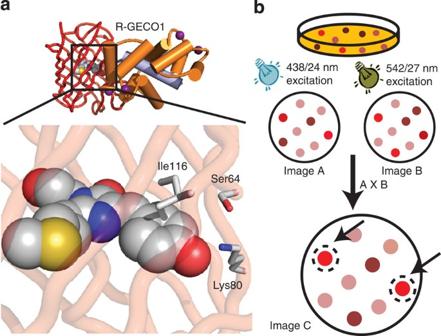Figure 1: Structure of R-GECO1 and screening scheme for REX-GECO. (a) Overall structure of R-GECO1 (PDB ID 4I2Y) and zoom in on its chromophore. The side chains of three proximal residues, Ser64, Lys80 and Ile116, are shown in stick format9. Residue numbering is consistent with the crystal structure of G-CaMP2 (PDB ID 3EVR)6. (b) Screening scheme to identify excitation ratiometric red fluorescent variants.E. colicolonies expressing REX-GECO variants were illuminated using either 438/24 nm or 542/27 nm light, and a red fluorescent image using 609/57 nm filter was acquired. The two resulting images were then multiplied to generate a third image in which colonies with strong moderate to strong intensity under both illumination conditions had the highest combined intensity. These colonies were selected for further testing. Figure 1: Structure of R-GECO1 and screening scheme for REX-GECO. ( a ) Overall structure of R-GECO1 (PDB ID 4I2Y) and zoom in on its chromophore. The side chains of three proximal residues, Ser64, Lys80 and Ile116, are shown in stick format [9] . Residue numbering is consistent with the crystal structure of G-CaMP2 (PDB ID 3EVR) [6] . ( b ) Screening scheme to identify excitation ratiometric red fluorescent variants. E. coli colonies expressing REX-GECO variants were illuminated using either 438/24 nm or 542/27 nm light, and a red fluorescent image using 609/57 nm filter was acquired. The two resulting images were then multiplied to generate a third image in which colonies with strong moderate to strong intensity under both illumination conditions had the highest combined intensity. These colonies were selected for further testing. Full size image Optimization of REX-GECO0.1 for improved function REX-GECO0.1’s fluorescence brightness and maturation rate, in the context of Escherichia coli colonies, were greatly reduced compared with R-GECO1. To engineer a variant with brighter fluorescence and a larger response to Ca 2+ , we applied both rational design and directed evolution. Based on our previous experience, the linker between M13 and the cpFP domain has an important role in the protein-folding efficiency and response to Ca 2+ (refs 10 , 11 ). In an effort to identify the optimal composition of this linker, we created a library by fully randomizing linker positions 60 and 61 (Pro and Val, respectively, in REX-GECO0.1). Screening of this library for bright long Stokes shift red fluorescence led to the identification of a variant with mutations Pro60Arg and Val61Trp (REX-GECO0.2). REX-GECO0.2 showed approximately threefold improved fluorescence brightness and improved maturation rate in Escherichia coli relative to REX-GECO0.1, while retaining a similar excitation ratio change on binding Ca 2+ . To further optimize REX-GECO0.2, we turned to a directed evolution strategy that involved multiple rounds of library creation by random mutagenesis and screening by fluorescence imaging of bacterial colonies. After each round the brightest clones were cultured, purified and subjected to a secondary screen in microplate format to determine their Ca 2+ response. A mixture of the 4–8 variants with the brightest fluorescence and largest responses to Ca 2+ was used as the template for the next round of library creation by random mutagenesis. For the first six rounds of this procedure, we screened libraries only on the basis of the brightness of their long Stokes shift red fluorescence in colonies. For the last two rounds of directed evolution, we switched to screening for proteins that exhibited a combination of bright long Stokes shift and short Stokes shift (excitation at 542/27 nm and emission 609/57 nm) fluorescence ( Fig. 1b ). The end products of these eight rounds of directed evolution were two improved variants: REX-GECO0.9 and REX-GECO1 with 15 and 14 mutations, respectively, relative to R-GECO1 ( Fig. 2a ; Supplementary Figs 1 and 2a ; Supplementary Table 1 ). 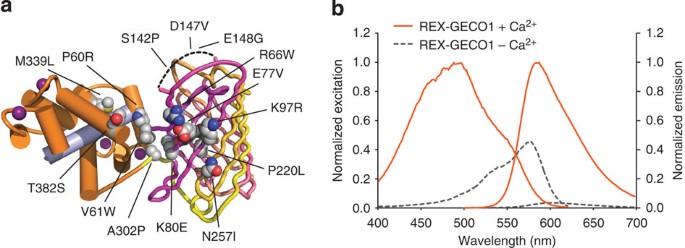Figure 2: Structural model and excitation, emission spectra of REX-GECO1. (a) Model of REX-GECO1, showing location of substitutions relative to R-GECO1 (PDB ID 4I2Y)9. Residue numbering is consistent with the crystal structure of G-CaMP2 (PDB ID 3EVR)6. (b) Excitation and emission spectra of REX-GECO1 both in the presence and absence of Ca2+. Figure 2: Structural model and excitation, emission spectra of REX-GECO1. ( a ) Model of REX-GECO1, showing location of substitutions relative to R-GECO1 (PDB ID 4I2Y) [9] . Residue numbering is consistent with the crystal structure of G-CaMP2 (PDB ID 3EVR) [6] . ( b ) Excitation and emission spectra of REX-GECO1 both in the presence and absence of Ca 2+ . Full size image In vitro characterization of REX-GECOs Systematic in vitro characterization of REX-GECO0.9 and REX-GECO1 revealed that these two proteins exhibit very similar spectral properties and differ primarily in their respective affinities for Ca 2+ . Specifically, REX-GECO1 ( K d =240 nM, k off =1.7 s −1 ) has a higher affinity for Ca 2+ than REX-GECO0.9 ( K d =680 nM, k off =3.2 s −1 ) ( Supplementary Fig. 3a,b ; Supplementary Table 2 ). Shared properties of the two proteins include excitation and emission maxima of 575 and 600 nm, respectively, in the Ca 2+ -free state. Once bound to Ca 2+ , these maxima shift to 480 and 585 nm, respectively ( Fig. 2b ; Supplementary Fig. 2b ; Supplementary Table 2 ). Both REX-GECOs showed a strong two-photon excitation peak at 910 nm ( Supplementary Fig. 3c,d ). Absorbance spectra with and without Ca 2+ are consistent with the fluorescence spectra ( Supplementary Fig. 3e,f ), but also reveal the presence of an additional non-excitable absorption peak at 450 nm in the Ca 2+ -free state. This peak likely corresponds to a population of the phenol form of the chromophore that is unable to undergo ESPT and instead undergoes excited state relaxation via a non-radiative pathway. REX-GECO0.9 and REX-GECO1 exhibit 70- and 100-fold maximal ratio changes, respectively, at physiological pH. These ratio changes decrease substantially at lower pH values, with apparent p K a s of 6.2 and 6.5, respectively ( Supplementary Fig. 3g,h ; Supplementary Table 2 ). Illumination with a 405 nm laser at 1,200 mW cm −2 induced a transient change of absorbance in the Ca 2+ -free state of both REX-GECO0.9 and REX-GECO1 ( Supplementary Fig. 3i,j ). This photoactivation phenomenon is drastically decreased in the Ca 2+ -bound state ( Supplementary Fig. 3k,l ). Owing to its higher Ca 2+ affinity, which we empirically found to be associated with better performance in neurons, REX-GECO1 is our preferred variant for imaging applications. Live cell performance of REX-GECO1 To explore the utility of REX-GECO1 for Ca 2+ imaging, we expressed it in cultured human cells, dissociated rat hippocampal pyramidal neurons, and organotypic rat hippocampal slices and performed a variety of intensiometric (one- and two-photon excitation) and ratiometric (one-photon) imaging experiments. Initial experiments with HeLa cells expressing REX-GECO1 revealed 13±5-fold intensity changes (fluorescence intensity for excitation at 472/30 nm and emission at 622/18 nm), and 36±19-fold ( n =36 cells) excitation ratio changes (ratio=fluorescence intensity for excitation at 472/30 nm with emission at 622/18 nm divided by fluorescence intensity from excitation at 620/60 nm with emission at 700/75 nm) on treatment with histamine ( Supplementary Fig. 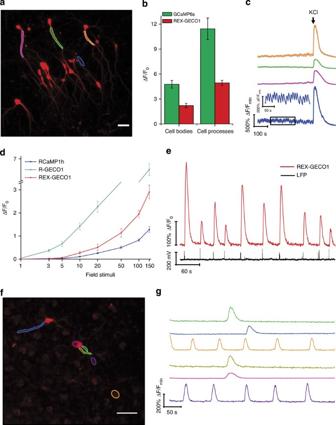Figure 3: Confocal imaging of REX-GECO1 in neurons and glial cells in organotypic brain slices. (a) An average intensity projection of a 3D Z-stack of images acquired for an organotypic rat hippocampal brain slice in which neurons are expressing REX-GECO1 under the synapsin I promoter. Scale bar represents 30 μm. (b) Comparison of REX-GECO1 and GCaMP6s in organotypic hippocampal brain slices. Response shown owing to theophylline excitation of brain slices transfected with REX-GECO1 or GCaMP6s (cell bodies: 2.2±0.5 and 4.8±0.9-fold, respectively,P<0.001; cell processes: 4.9±0.6 and 11±3-fold, respectively,P<0.001). Data are mean fluorescence change (ΔF/F0)±s.d. (c) Fluorescence versus time traces for single cells as indicated in (a) on treatment with 10 mM theophylline, followed by 30 mM KCl. The trace colour corresponds to regions marked in (a). Inset: Zoom in on theophylline-induced fluorescence oscillations as marked by black borderline. (d) Characterization of REX-GECO1 (n=8 cells), R-GECO1 (n=7 cells), and RCaMP (n=7 cells) in cultured organotypic hippocampal slices. Data points are mean fluorescence change (ΔF/F0)±s.d. in response to 100 Hz field stimulation induced action potential trains. (e) Simultaneous recording of both REX-GECO1 fluorescence change (ΔF/F0) (red) and the local field potential (LFP) (black) in response to theophylline treatment in rat organotypic hippocampal brain slice. (f) An average intensity projection of a 3D Z-stack of glial cells expressing REX-GECO1 under CMV promoter in an organotypic rat hippocampal slice. Scale bar represents 30 μm. (g) Glutamate-induced Ca2+oscillations in glial cell bodies and processes as indicated in (f). Colours of the traces correspond to the colors of the regions marked in (f). 4a ; Supplementary Table 3 ). When imaged using two-photon microscopy (excitation at 910 nm with a laser power of 0.2 W (180 μW, when measured at the front of the objective), and emission at 642.5/75 nm), REX-GECO1 photobleached to 50% of its initial fluorescence after 294 s of continuous illumination ( Supplementary Fig. 4b ). On treatment of cells with histamine, REX-GECO1 showed a 5±2-fold ( n =30 cells) intensity change ( Supplementary Fig. 4c ), which is consistent with our results from one-photon excitation ( Supplementary Table 3 ). To compare the fluorescent brightness of REX-GECO1 and R-GECO1 (ref. 11 ) under two-photon excitation, transfected HeLa cells (treated with CaCl 2 (10 mM) and ionomycin (5 μM)) were imaged by two-photon microscopy with excitation at 910 and 1,040 nm. When excited at 910 nm (laser power of 0.1 W (90 μW, when measured at the front of the objective), with emission at 642.5/75 nm), HeLa cells expressing REX-GECO1 showed high red fluorescence intensity ( Supplementary Fig. 4d ), whereas the R-GECO1-expressing cells were barely detectable ( Supplementary Fig. 4e ). Reasoning that 910 nm is not the optimal wavelength for two-photon excitation of R-GECO1, we also used 1,040 nm and the maximal laser power of 0.61 W (1,200 μW, when measured at the front of the objective) with emission at 642.5/75 nm. Even at this longer wavelength, a robust red fluorescent signal was not observed for R-GECO1 ( Supplementary Fig. 4f ). Overall, REX-GECO1 showed significantly higher brightness compared with R-GECO1 when imaged with two-photon excitation. Next, we investigated the performance of REX-GECO1 in dissociated rat hippocampal neurons. REX-GECO1 has a K d of 240 nM, making it suitable for detection of neuronal Ca 2+ oscillations (typically from ∼ 50 to 250 nM) [25] . In this context, neurons expressing REX-GECO1 gave more than twofold ratio changes for spontaneous Ca 2+ changes using the same one-photon imaging conditions used for HeLa cells ( Supplementary Fig. 4g,h ). To compare the performance of REX-GECO1 with the current RFP-based Ca 2+ indicators, we expressed REX-GECO1, RCaMP1h [9] and R-GECO1 (ref. 11 ) in neurons in organotypic hippocampal brain slices by ex vivo electroporation. After 3–6 days, transfected neurons were imaged following field stimulation using an extracellular electrode. Peak Δ F / F 0 was extracted from fluorescence signals of individual neurons and the average response to each field stimulus was plotted for each indicator ( Fig. 3d ). REX-GECO1 showed detectable fluorescence response (3±1%) following a minimum of three field stimuli and reaching a maximum response of 291±27% following 150 field stimuli. RCaMP1h started to show fluorescence response following a minimum of five field stimuli and reached a maximum response of 128±12% following 150 stimuli. R-GECO1 showed fluorescence response to single-field stimulation (4±1%) and reached a maximum response of 656±25% following 150 field stimuli. Figure 3: Confocal imaging of REX-GECO1 in neurons and glial cells in organotypic brain slices. ( a ) An average intensity projection of a 3D Z-stack of images acquired for an organotypic rat hippocampal brain slice in which neurons are expressing REX-GECO1 under the synapsin I promoter. Scale bar represents 30 μm. ( b ) Comparison of REX-GECO1 and GCaMP6s in organotypic hippocampal brain slices. Response shown owing to theophylline excitation of brain slices transfected with REX-GECO1 or GCaMP6s (cell bodies: 2.2±0.5 and 4.8±0.9-fold, respectively, P <0.001; cell processes: 4.9±0.6 and 11±3-fold, respectively, P <0.001). Data are mean fluorescence change (Δ F / F 0 )±s.d. ( c ) Fluorescence versus time traces for single cells as indicated in ( a ) on treatment with 10 mM theophylline, followed by 30 mM KCl. The trace colour corresponds to regions marked in ( a ). Inset: Zoom in on theophylline-induced fluorescence oscillations as marked by black borderline. ( d ) Characterization of REX-GECO1 ( n =8 cells), R-GECO1 ( n =7 cells), and RCaMP ( n =7 cells) in cultured organotypic hippocampal slices. Data points are mean fluorescence change (Δ F / F 0 )±s.d. in response to 100 Hz field stimulation induced action potential trains. ( e ) Simultaneous recording of both REX-GECO1 fluorescence change (Δ F / F 0 ) (red) and the local field potential (LFP) (black) in response to theophylline treatment in rat organotypic hippocampal brain slice. ( f ) An average intensity projection of a 3D Z-stack of glial cells expressing REX-GECO1 under CMV promoter in an organotypic rat hippocampal slice. Scale bar represents 30 μm. ( g ) Glutamate-induced Ca 2+ oscillations in glial cell bodies and processes as indicated in ( f ). Colours of the traces correspond to the colors of the regions marked in ( f ). Full size image We further tested the performance of REX-GECO1 in hippocampal neurons and glial cells in rat organotypic hippocampal slices using two different plasmids with different promoters ( Fig. 3a,f ). Human synapsin I promoter was used for preferential expression of REX-GECO1 in neurons [26] , [27] ( Supplementary Fig. 5a ). A cytomegalovirus (CMV) promoter was used to drive preferential expression of REX-GECO1 in glial cells [28] ( Supplementary Fig. 5b ). Hippocampal slices were transiently transfected by ex vivo electroporation, and were cultured for 8–12 days (5–7 days post transfection). Expression of REX-GECO1 in the cytoplasm of neural cells led to visualization of both the cell bodies and processes ( Figs 3a,f and 4a ; Supplementary Movies 1,2 and 3 ). Transfected cells were healthy on the basis of their morphology ( Supplementary Fig. 5 ) and responsive as they showed expected pharmacologically induced Ca 2+ rises. During imaging, we did notice a few intracellular puncta in the cell bodies of some neurons and glial cells, but this did not affect the health or response of those cells. 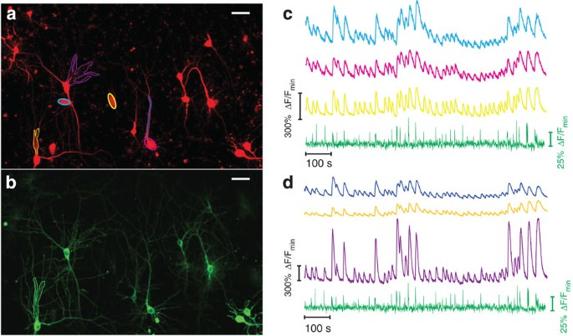Figure 4: One-photon confocal dual-color imaging of REX-GECO1 co-expressed with a green glutamate indicator (iGluSnFR) in organotypic rat hippocampal slices. (a) An average intensity projection of a 3D Z-stack of neurons expressing REX-GECO1 under synapsin I promoter in a hippocampal slice, Scale bar represents 30 μm. (b) An average intensity projection of a 3D Z-stack of the neurons in (a) expressing iGluSnFR under synapsin I promoter in a hippocampal slice, Scale bar represents 30 μm. (c,d) Simultaneous imaging of theophylline-induced Ca2+oscillations and glutamate transients in (c) neuron cell bodies and (d) neuron processes as highlighted in (a) and (b). Colours of the traces correspond to the colours of the highlighted regions. The glutamate signal is shown in green in both graphs. Figure 4: One-photon confocal dual-color imaging of REX-GECO1 co-expressed with a green glutamate indicator (iGluSnFR) in organotypic rat hippocampal slices. ( a ) An average intensity projection of a 3D Z-stack of neurons expressing REX-GECO1 under synapsin I promoter in a hippocampal slice, Scale bar represents 30 μm. ( b ) An average intensity projection of a 3D Z-stack of the neurons in ( a ) expressing iGluSnFR under synapsin I promoter in a hippocampal slice, Scale bar represents 30 μm. ( c , d ) Simultaneous imaging of theophylline-induced Ca 2+ oscillations and glutamate transients in ( c ) neuron cell bodies and ( d ) neuron processes as highlighted in ( a ) and ( b ). Colours of the traces correspond to the colours of the highlighted regions. The glutamate signal is shown in green in both graphs. Full size image When expressed in neurons, REX-GECO1 exhibited bright baseline fluorescence when excited by a 543 nm laser. For imaging of dynamic Ca 2+ oscillations, we switched to a 488 nm laser for excitation and used theophylline (10 mM) to pharmacologically excite neurons in organotypic brain slices. Theophylline, at low millimolar concentration, blocks both adenosine and GABA A receptors and has been shown to evoke sustained rhythmic seizure-like activities in different neural networks including hippocampal neurons [29] , [30] , [31] , [32] , [33] . Indeed, on treatment with theophylline, REX-GECO1 (under synapsin I promoter) successfully detected neuronal Ca 2+ transients and oscillations with large fluorescence intensity changes (cell bodies: 2.2±0.5-fold, n =8 cells; cell processes: 4.9±0.6-fold, n =9 cells) ( Figs 3b,c and 4c,d ; Supplementary Movie 1 ). We placed an extracellular electrode in close proximity to the cells being imaged to simultaneously record the local field potential (LFP) in response to theophylline treatment. Simultaneous recordings of the LFP and REX-GECO1 fluorescence showed that REX-GECO1 was able to faithfully report neural activity in response to theophylline treatment ( Fig. 3e ). Under identical conditions, GCaMP6s [7] , one of the most highly optimized GFP-derived Ca 2+ indicators, exhibits fluorescence changes in response to theophylline (cell bodies: 4.8±0.9-fold, n =5 cells; cell processes: 11±3-fold, n =5 cells) that are approximately double that of REX-GECO1 ( Fig. 3b ). Depolarization of REX-GECO1-expessing neurons with 30 mM KCl, which activates voltage-gated Ca 2+ channels to promote Ca 2+ influx [34] , [35] , increased fluorescence intensity by 12±3-fold ( n =8 cells). Bath application of glutamate was used to evoke Ca 2+ rises in hippocampal glial cells expressing REX-GECO1 (under the CMV promoter). Activation of the glutamate receptors on glial cells leads to an increase in intracellular Ca 2+ levels mostly due to ‘metabotropic’ release from endoplasmic reticulum [36] , [37] , [38] . This Ca 2+ increase has been described as oscillatory waves of elevated intracellular Ca 2+ concentration spreading across glial cells [39] , [40] , including those of the rat hippocampus [41] . REX-GECO1 successfully detected Ca 2+ rises in both glial cell bodies (2±1-fold, n =4 cells) and their processes (3.7±0.9-fold, n =10 cells) with sufficient spatial and temporal resolution to allow us to visualize Ca 2+ waves across the cells as described previously ( Fig. 3f,g ; Supplementary Movie 2 ). Overall, REX-GECO1 showed robust responses to the activities of neural cells. REX-GECO1 for dual-colour imaging in rat organotypic slice We next investigated the utility of REX-GECO1 in multicolour imaging together with a second genetically encoded indicator. As REX-GECO1 has a Ca 2+ -dependent excitation peak at 480 nm, we reasoned that it could also be used as an intensiometric red Ca 2+ indicator with a large Stokes shift, and thereby combined with an intensiometric green indicator for multicolour imaging using a single excitation wavelength. To demonstrate this, we set out to image both Ca 2+ and glutamate responses in organotypic rat hippocampal slice cultures. We reasoned that because pyramidal hippocampal neurons are glutamatergic [42] , one would be able to simultaneously detect Ca 2+ transients and glutamate release when they are excited. We co-expressed REX-GECO1 in the cytosol and a green glutamate indicator, iGluSnFR [43] , on the plasma membrane of neurons using a synapsin I promoter for both indicators ( Fig. 4a,b ) and used theophylline to induce seizure-like activity in hippocampal neurons as described above. Using one-photon excitation at 488 nm, we successfully recorded simultaneous glutamate release (green channel) and Ca 2+ transients (red channel). REX-GECO1 revealed Ca 2+ rises in both the cell bodies and processes ( Fig. 4c,d ; Supplementary Movie 3 ) of hippocampal neurons with large signal magnitude (cell bodies: 2.2±0.5-fold, n =7 cells; cell processes: 4.9±0.6-fold, n =7 cells). In neurons that were only transfected with REX-GECO1 but not iGluSnFR, we did not observe any crosstalk from REX-GECO1 into the green channel ( Supplementary Fig. 6 ). A short lasting ( ∼ 0.5 s) increase in glutamate ( Supplementary Movie 4 ), as released from surrounding neurons [44] , was followed by a longer ( ∼ 10–20 s) Ca 2+ rise in neurons expressing both REX-GECO1 and iGluSnFR, indicating that the Ca 2+ influx was induced by glutamate. Similar results were obtained using two-photon excitation at 940 nm for both REX-GECO1 and iGluSnFR ( Fig. 5 ; Supplementary Movie 5 ). Overall, these results demonstrate that REX-GECO1 can be combined with GFP-based indicators to create new opportunities for simultaneous multicolour one- and two-photon imaging. 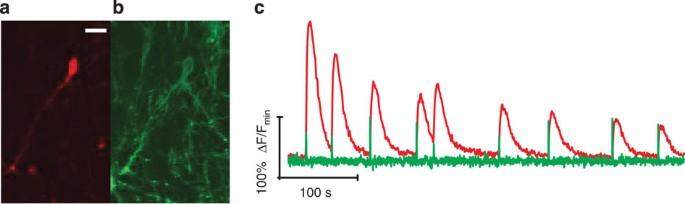Figure 5: Two-photon dual-color imaging of neurons co-expressing REX-GECO1 and iGluSnFR in organotypic rat hippocampal brain slices. (a) A neuron expressing cytoplasmic REX-GECO1 under synapsin I promoter in a hippocampal slice (emission 605–680 nm), Scale bar represents 20 μm. (b) The same neuron as in (a) co-expressing iGluSnFR on the plasma membrane (emission 460–500 nm). (c) Theophylline-induced Ca2+(red) and glutamate (green) transients and oscillations in the neuron in (a) and (b) excited at 940 nm. Figure 5: Two-photon dual-color imaging of neurons co-expressing REX-GECO1 and iGluSnFR in organotypic rat hippocampal brain slices. ( a ) A neuron expressing cytoplasmic REX-GECO1 under synapsin I promoter in a hippocampal slice (emission 605–680 nm), Scale bar represents 20 μm. ( b ) The same neuron as in ( a ) co-expressing iGluSnFR on the plasma membrane (emission 460–500 nm). ( c ) Theophylline-induced Ca 2+ (red) and glutamate (green) transients and oscillations in the neuron in ( a ) and ( b ) excited at 940 nm. Full size image REX-GECO1 for in vivo imaging One of the most powerful applications of genetically encoded Ca 2+ indicators is minimally invasive monitoring of neuronal activity in vivo . We used DNA electroporation to drive expression of REX-GECO under the CMV promoter, co-expressed with EGFP, in the eye and optic tectum of albino Xenopus laevis tadpoles ( Fig. 6a ). Animals were imaged by two-photon microscopy at least 2 days after electroporation to allow sufficient protein expression. We first used an ex vivo isolated brain preparation to the monitor Ca 2+ elevation in optic tectal neurons co-expressing REX-GECO0.9 and EGFP in response to pharmacological activation of NMDA ( N -methyl-D-aspartate) type ionotropic glutamate receptors ( Fig. 6b ). Bath application of 20 μM NMDA resulted in a robust increase in the ratio of red to green fluorescence in these cells (2.2±0.4-fold, n =6 cells). We next tested whether REX-GECO1 could be used to detect neuronal responses to more physiological stimuli, by presenting brief pulses of light to activate neurons in the visual system of the intact animal. Neurons in the optic tectum, the primary visual area in the tadpole brain, are readily distinguishable from radial glial cells on the basis of their position and morphology. 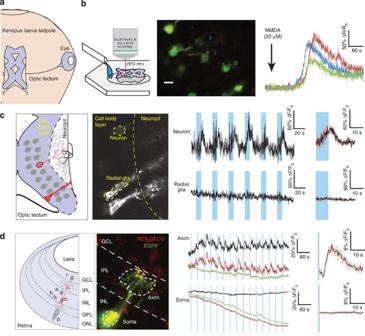Figure 6:Ex vivoandin vivotwo-photon microscopy of REX-GECO responses to pharmacological and visual stimulation in the retinotectal system ofXenopus laevistadpoles. (a) The eye projects visual inputs to the contralateral optic tectum in the tadpole (OB, olfactory bulb; DiE, diencephalon; E, eye; OT, optic tectum; and HB, hindbrain). (b) An isolated brain preparation with tectal neurons co-expressing REX-GECO0.9 (red) and EGFP (green) imaged at 910 nm responding to bath application of 20 μM NMDA for the three cells indicated.Middle: two-photon z-stack projection. (c)In vivotectal neuron co-expressing REX-GECO1 and EGFP exhibits Ca2+transients in response to 10 s light flashes to the eye (blue bars). Radial glia is unresponsive. Regions of interest drawn for the cells analyzed.Right: average of visually evoked responses (black)±s.e.m. (red). (d) Non-spiking retinal bipolar cell co-electroporated with REX-GECO1 (red) and EGFP (green) shows light-evoked Ca2+elevations in the neuropil but not in the cell soma. (ONL—outer nuclear layer; OPL—outer plexiform layer; INL—inner nuclear layer; IPL—inner plexiform layer; GCL—ganglion cell layer; p.—photoreceptor; h.—horizontal cell; b.—bipolar cell; a.—amacrine cell; and r.—retinal ganglion cell). Plots of somatic and axonal ΔF/F0for REX-GECO1 (red) and EGFP (green) in response to 2 s light flashes (blue bars). The black trace is REX-GECO1 with EGFP ΔF/F0subtracted.Right: averaged responses of the bipolar cell subdomains to light flashes. Figure 6c shows an example of REX-GECO1 fluorescence changes in the cell body of a tectal neuron in response to 10-s light flashes presented to the contralateral eye (max Δ F / F 0 of mean response=71%). As expected, the neighbouring radial glia cell showed no light-evoked response above noise for this experiment, despite higher levels of expression. In the retina, light modulates glutamate release from photoreceptors onto bipolar cells, driving a change in their membrane potential. Unlike tectal neurons, bipolar cells do not fire action potentials, but instead rely on voltage-dependent Ca 2+ influx at their axon terminals to continuously modulate neurotransmitter release. Consequently, 1-s light flashes evoked small but consistent increases in REX-GECO1 fluorescence in the axon terminals (max Δ F / F 0 of mean response=10.3%) but not at the bipolar cell soma (max Δ F / F 0 of mean signal=0.7%) ( Fig. 6d ). EGFP fluorescence did not respond to visual stimulation, making it useful for correcting for gradual specimen drift that can be a common problem when imaging in the intact animal. These results demonstrate that REX-GECO1 can be used to detect physiological subcellular Ca 2+ changes in neurons in vivo . Figure 6: Ex vivo and in vivo two-photon microscopy of REX-GECO responses to pharmacological and visual stimulation in the retinotectal system of Xenopus laevis tadpoles. ( a ) The eye projects visual inputs to the contralateral optic tectum in the tadpole (OB, olfactory bulb; DiE, diencephalon; E, eye; OT, optic tectum; and HB, hindbrain). ( b ) An isolated brain preparation with tectal neurons co-expressing REX-GECO0.9 (red) and EGFP (green) imaged at 910 nm responding to bath application of 20 μM NMDA for the three cells indicated. Middle : two-photon z-stack projection. ( c ) In vivo tectal neuron co-expressing REX-GECO1 and EGFP exhibits Ca 2+ transients in response to 10 s light flashes to the eye (blue bars). Radial glia is unresponsive. Regions of interest drawn for the cells analyzed. Right : average of visually evoked responses (black)±s.e.m. (red). ( d ) Non-spiking retinal bipolar cell co-electroporated with REX-GECO1 (red) and EGFP (green) shows light-evoked Ca 2+ elevations in the neuropil but not in the cell soma. (ONL—outer nuclear layer; OPL—outer plexiform layer; INL—inner nuclear layer; IPL—inner plexiform layer; GCL—ganglion cell layer; p.—photoreceptor; h.—horizontal cell; b.—bipolar cell; a.—amacrine cell; and r.—retinal ganglion cell). Plots of somatic and axonal Δ F / F 0 for REX-GECO1 (red) and EGFP (green) in response to 2 s light flashes (blue bars). The black trace is REX-GECO1 with EGFP Δ F / F 0 subtracted. Right : averaged responses of the bipolar cell subdomains to light flashes. Full size image By utilizing rational design and directed evolution, we have developed a red fluorescent Ca 2+ indicator, REX-GECO1, with in vitro intensiometric changes of 35-fold (480 nm excitation) and ratiometric changes of 100-fold (585 nm excitation/480 nm excitation). We have demonstrated the versatility of REX-GECO1 by imaging of Ca 2+ dynamics with one-photon (480 nm) and two-photon ( ∼ 910–940 nm) excitation in a variety of cell types and contexts, including organotypic rat hippocampal slices and tectal neurons in the tadpole brain. REX-GECO1 also enables simultaneous dual-colour imaging together with a GFP-based fluorescent probe, as we have demonstrated by simultaneous imaging of both Ca 2+ and glutamate in both one- and two-photon modalities. On the basis of empirical testing of performance in neurons, REX-GECO1 was found to give superior performance to REX-GECO0.9, our second most promising variant. We attribute the improved performance of REX-GECO1 to its higher Ca 2+ affinity ( K d =240 nM) relative to REX-GECO0.9 ( K d =680 nM). The differences in Ca 2+ affinity are likely due to the Glu138Val mutation in REX-GECO0.9, which is on the surface of the cpFP domain and has its side chain directed towards the second EF-hand of CaM. The Glu138Val substitution likely alters key interactions involved in communicating the Ca 2+ -dependent conformational change of CaM into a change in the chromophore environment. We suspect that REX-GECO0.9 could prove more useful than REX-GECO1 in cell types with a higher basal Ca 2+ concentration. Our success at engineering REX-GECO1 from its R-GECO1 progenitor emphasizes the critical nature of the interaction between the side chain of Lys80 and the phenolate moiety of the R-GECO1 chromophore, as observed in the crystal structure (PDB ID 4I2Y) [9] . We presume that, in R-GECO1, the Ca 2+ -dependent interaction of CaM and M13 acts to reorganize the interface with the FP domain and position the positively charged amine group of Lys80 in close proximity to the phenol group of the chromophore. The electrostatic interaction serves to decrease the p K a of the chromophore, thereby increasing the proportion of the protein in the bright fluorescent phenolate form [11] . In the absence of Ca 2+ , the conformation of the Lys80 side chain is presumably less restrained and it is directed away from the chromophore and towards the bulk solvent. This mechanism is similar to that proposed for GCaMP, in which the protonation state of the chromophore is modulated by interaction with Arg377 of CaM [6] . As described in this work, the dramatically modified spectral characteristics bestowed on the protein by the Lys80Glu substitution are the defining feature of the REX-GECO series of variants. By analogy with the mechanism of R-GECO1, Ca 2+ binding to REX-GECO1 leads to a positioning of the negatively charged carboxylate moiety close to the phenol group of the chromophore. As the p K a of the carboxylate is lower than that of the chromophore, this interaction is expected to stabilize the neutral phenol. On excitation, the p K a of the chromophore drops below that of the carboxylate and ESPT produces the carboxylic acid and the red fluorescent phenolate form of the chromophore. In the Ca 2+ -free state, REX-GECO1 exists as a mixture of both the phenol and phenolate forms of the chromophore. Although the phenolate form does produce red fluorescence if excited, the phenol form is incapable of ESPT and therefore non-fluorescent ( Fig. 2b ). This result is consistent with our proposed mechanism, and indicates that, just like with Lys80 of R-GECO1, the side chain of Glu80 is directed away from the chromophore and exposed to the bulk solvent in the absence of Ca 2+ . Notably, the self-contained fluorescence modulation mechanisms of R-GECO1 and REX-GECO1 (that is, not dependent on specific interactions with CaM, as is the case for GCaMP) make the cpFP domains of these proteins particularly promising templates for combination with other sensing domains to engineer new types of genetically encoded reporters. Most GCaMP-type indicators, and all of the red fluorescent ones reported to date, respond to Ca 2+ with an intensiometric response. However, for many applications it is desirable to have a ratiometric response where an increase in intensity at one wavelength is associated with a decrease at another. Indeed, a ratiometric response is inherent to all Förster resonance energy transfer-based Ca 2+ indicators with a fluorescent acceptor [3] , [45] , and excitation and emission ratiometric green fluorescent GCaMP-type indicators have been reported [4] , [11] . As we have demonstrated in this work, REX-GECO1 responds to Ca 2+ with an excitation ratiometric response. However, we did find that the broad excitation peak associated with the Ca 2+ -bound state, together with the very short 3 nm wavelength difference between the excitation maximum for the Ca 2+ -free state and the emission maximum for the Ca 2+ -bound state, introduce some technical challenges for ratiometric imaging. To achieve satisfactory ratiometric imaging, we resorted to using a relatively long wavelength Cy5 filter set (excitation at 620/60 nm with emission at 700/75 nm) for the Ca 2+ -free state. Although this filter set is not an optimal match for the Ca 2+ -free REX-GECO1 spectral profile, it did minimize excitation of the Ca 2+ -bound state of the chromophore while still providing sufficient fluorescence intensity. An additional benefit of the ratiometric fluorescence response of REX-GECO1 is that it facilitates the identification of transfected cells in their resting state. When imaging sparsely transfected organotypic slice cultures, we found that REX-GECO1 exhibits dim baseline fluorescence with 488-nm laser excitation but bright red fluorescence with 543-nm laser excitation. Although we observed a transient change of absorbance in both purified REX-GECO0.9 and REX-GECO1 proteins on strong (1,200 mW cm −2 ) violet-light illumination ( Supplementary Fig. 3i-l ), this photoactivation phenomenon is unlikely to occur under typical imaging conditions. In our fluorescence imaging of REX-GECO, we have not observed any artifactual differences in fluorescent intensity between the first and subsequent acquired images, as would be expected if the initial illumination was inducing photoconversion. The availability of REX-GECO1 provides new possibilities for one- and two-photon Ca 2+ imaging using genetically encoded indicators with high sensitivity. We expect that REX-GECO1 will have broad appeal as the preferred Ca 2+ indicator for use in combination with any of the plethora of GFP-based probes and indicators currently available. Engineering and screening of REX-GECO For the engineering of REX-GECO, R-GECO1 in pTorPE [11] was used as a template. Point mutations to R-GECO1 were performed using QuikChange II Site-Directed Mutagenesis Kit (Agilent Technologies). Random mutagenesis was generated by error-prone polymerase chain reaction (PCR) amplification. In the first generation library, the codon for residue 64 was mutated to BMM (where B=guanine and cytosine and thymine and M=adenine and cytosine; encoding Ala, Asp, Gln, Glu, His, Pro, Ser and Tyr), the codon for residue 80 was mutated to VAN (where V=guanine and adenine and cytosine and A=adenine and N=guanine and adenine and thymine and cytosine; encoding Asn, Asp, Gln, Glu, His, and Lys) and the codon for residue 116 was mutated to VHM (where H=adenine and thymine and cytosine; encoding Ala, Asn, Asp, Gln, Glu, His, Ile, Leu, Lys, Met, Pro, Thr, and Val). For REX-GECO variants screening, the imaging system used has been described in detail [46] . PTorPE plasmids containing REX-GECO variants were electroporated into E. coli strain DH10B (Invitrogen). These E. coli were then cultured on 10-cm Lysogeny broth (LB)-agar Petri dishes supplemented with 400 μg ml −1 ampicillin (Sigma) and 0.0004% (wt/vol) L -arabinose (Alfa Aesar) at 37 °C overnight. During screening, a 609/57 nm emission filter was used to capture the fluorescence emission. Two images, image A and image B, were captured by using excitation filter of 438/24 nm or 542/27 nm to illuminate E. coli colonies expressing REX-GECO variants on Petri dishes. These two images were then multiplied to generate a third image C. Colonies that showed the highest 0.1% emission intensities in image C were picked and cultured in 4 ml liquid LB with 100 μg ml −1 ampicillin and 0.0016% (wt/vol) L -arabinose at 37 °C overnight. Proteins were then extracted from the liquid LB culture and subjected to a secondary screen by using a Safire2 fluorescence microplate reader (Tecan). Characterization of REX-GECO1 REX-GECO1 proteins were purified as previously described [11] . To measure the fluorescence and absorbance spectra of REX-GECO, a QuantaMaster spectrofluorometer (Photon Technology International), and a DU-800 UV-visible spectrophotometer (Beckman) were used, respectively. REX-GECO1’s extinction coefficient ( ɛ ), quantum yield (Φ), p K a and K d were determined as previously described [11] with mCherry and LSS-mKate2 serving as standards. A SX20 stopped-flow spectrometer (Applied Photophysics) was used to measure k off . Briefly, Protein samples with 10 μM CaCl 2 (in 10 mM MOPS, 100 mM KCl pH 7.2) were rapidly mixed with a solution with 10 mM EGTA (in 10 mM MOPS, 100 mM KCl pH 7.2) at room temperature. The k off was determined by fitting the fluorescence decay curve to a single exponential equation. Each protein sample was measured five times, and the averaged value was taken as k off . For characterization of photoactivation of REX-GECOs, purified proteins were diluted to an absorbance value in the range of 0.1–0.5 in a buffered solution. Spectra were recorded using a UV–visible spectrometer (Agilent 8453 spectrophotometer) with or without illumination from a 150 mW (1,200 mW cm −2 ) 405 nm laser (Changchun New Industries Optoelectronics Tech.). Two-photon absorption spectra were measured using fluorescence femtosecond setup, described previously [21] . Briefly, it comprises a tunable parametric amplifier (550–2,000 nm) producing ∼ 100 fs pulses with 1 kHz repetition rate. Rhodamine B in methanol was used as a reference standard [47] for both the spectral shape and absolute cross section evaluations. The cross-sections were measured at 900, 1,000 and 1,130 nm. The quadratic power dependence of fluorescence signal was checked at several wavelengths across the spectrum. The concentration of proteins with matured chromophore was evaluated spectrophotometrically by using the extinction coefficients measured by alkaline denaturation method (see above) and presented in Supplementary Table 2 . Note that Supplementary Fig. 3 presents the effective two-photon cross-section weighted with the relative fractions of neutral (protonated), n (n) , and anionic (deprotonated), n (a) , forms: σ 2 ( λ )= n (n) σ 2 (n) ( λ )+ n (a) σ 2 (a) ( λ ), where σ 2 (n) ( λ ) and σ 2 (a) ( λ ) are the molecular two-photon absorption cross-sections of the neutral and anionic forms, respectively, and n (n) + n (a) =1. Plasmids for mammalian cell imaging For REX-GECO1 plasmid with a CMV promoter, template (REX-GECO1 in pTorPE [11] ) was cloned into a modified pcDNA3 plasmid by PCR as previously described [10] . This vector was used in one-photon, two-photon imaging of HeLa cells and one-photon imaging of dissociated rat hippocampal neurons. For REX-GECO1 plasmid with a human synapsin I promoter, template (REX-GECO1 in pTorPE) was cloned into an AAV2 plasmid flanked by restriction sites BamH1 and HindIII by PCR using following primers: BamH1_fw (5′-GAGGATCCACCATGGTCGACTCATCACGTC-3′) and HindIII_rv (5′-GCGATGAAGCTTCTACTTCGCTGTCATCATTTGTACAAACTCTTCGTAGTTT-3′). For iGluSnFR plasmid with a human synapsin I promoter, iGluSnFR (Addgene plasmid 41732) was used as a template and cloned into an AAV2 plasmid flanked by restriction sites BamH1 and HindIII by PCR using following primers: BamH1_iGlu_fw (5′-CGAGGATCCGCCACCATGGAGACAG ACACACTCCTGCTATGGGTAC-3′) and HindIII_iGlu_rv (5′-CCCTTATCATCCTCATCA TGCTTTGGCAGAAGAAGCCACGTTAGAAGCTTCGATCC-3′). For GCaMP6s R-GECO1 and RCaMP1h plasmid (with a human synapsin I promoter) used in comparison with REX-GECO1 in rat hippocampal organotypic brain slices, GCaMP6s (Addgene plasmid 40753), R-GECO1 and RCaMP1h (Addgene plasmid 42874) were used as a template and cloned into the same AAV2 plasmid, respectively. Cell culture HeLa cells (CCL2 line; ATCC) were cultured on collagen-coated 35-mm glass bottom dishes (Matsunami) until they reached 40–60% confluency. Transfection was performed by incubating HeLa cells with the mixture of 1 μg of plasmid DNA and 3 μl of Lipofectamine 2000 (Life Technologies) for 2 h. After incubation, the medium was exchanged to DMEM (supplemented with 10% fetal bovine serum (FBS; Sigma), 2 mM GlutaMax (Invitrogen) and penicillin-streptomycin) and the cells were incubated for 48 h at 37 °C in a CO 2 incubator. Before imaging, culture medium was changed to HEPES (25 mM) buffered Hanks’ balanced salt solution (HBSS). Dissociated E18 Sprague Dawley Hippocampal Cells in Hibernate EB Complete Media were purchased from BrainBits LLC. The cells were grown on ( In Vitro Scientific) 35 mm glass bottom dish containing NbActiv4 (BrainBits LLC) supplemented with 2% FBS, penicillin-G potassium salt (50 units ml −1 ), and streptomycin sulfate (50 μg ml −1 ). Half of the culture media is replaced every 4–5 days. Neuronal cells were transfected on day 7 with plasmids containing constructs of interest using Lipofectamine 2000. Transfection of rat hippocampal organotypic brain slices Horizontal brain slices (250 μm thickness) from a 0-day-old (P0) Sprague Dawley rat were generated in ice-cold HBSS containing 1.3 mM CaCl 2 and 1 mM MgSO 4 with a vibrating microtome (Leica VT1000S, Leica Microsystems, Richmond Hill, ON, Canada) as described previously [30] . All procedures were carried out in compliance with the guidelines of the Canadian Council for Animal Care and with the approval of the University of Alberta Animal Care and Use Committee for Health Science. Hippocampal regions were cut from horizontal brain slices and placed on a sterile 0.4-μm-pore-membrane cell culture insert (Millipore PICMORG50). The insert and slice were then placed in a Petri dish containing 1.5 ml of NbActiv4 (BrainBits) supplemented with 5% FBS, penicillin-G potassium salt (50 units ml −1 ), and streptomycin sulfate (50 μg ml −1 ). Slices are cultured at 37 °C and 5% CO 2 for 24 h before transfection by electroporation. The insert and slice are then placed directly above a Platinum Plate Petri dish electrode (CUY700-P2E, Nepa Gene, Japan) and the gap between the electrode and the membrane is filled with electroporation buffer (EB) (HBSS with 1.5 mM MgCl 2 and 10 mM D -glucose). Plasmids (pcDNA3.1, Life Technologies and AAV2 plasmid) for expression of the gene of interest are dissolved in EB at a concentration of 1 μg μl −1 and sufficient volume is added to just cover the slice. A square platinum electrode (CUY700-P2L, Nepa Gene, Japan) is then placed directly above the hippocampus slice and a power supply is used to apply five 20 V pulses (5 ms each, 1 Hz). The direction of electrical field is reversed and a second set of five pulses with the same settings is applied. The EB is carefully replaced with supplemented NbActiv4 and slices are returned to incubator at 37 °C with 5% CO 2 . Microscopes for fluorescence imaging Widefield imaging was performed on an inverted Nikon Eclipse Ti microscope equipped with a 200 W metal halide lamp (PRIOR Lumen), × 20 and × 40 objectives (Nikon), and a 16-bit QuantEM 512SC electron-multiplying charge-coupled device (CCD) camera (Photometrics). A filter set of 472/30 nm (excitation), 622/18 nm (emission) and 495 nm (dichroic) was used for long Stokes shift excitation. Another filter set of 620/600 nm (excitation), 700/75 nm (emission) and 666 nm (dichroic) was used for short Stokes shift excitation. For time-lapse imaging, HeLa cells were treated with 5 μM (final concentration) histamine, 4 mM EGTA (with 5 μM ionomycin) and 10 mM CaCl 2 (with 5 μM ionomycin) in chronological order. Regions of interest (ROIs) corresponding to visually identifiable and healthy cells (based on their morphology) were selected for analysis. For one-photon imaging, we used an upright FV1000 confocal microscope (OlympusCanada, Markham, ON, Canada) equipped with software (FluoView1000, Olympus Canada), a × 20 XLUMPlanF1 water immersion objective (numerical aperture (NA)=1.00), or a × 60 XLUMPlanF1 water immersion objective (NA=0.90), and connected to multi-line argon lasers (457, 488 and 515 nm) and HeNe lasers (543 and 633 nm) (Olympus Canada). For two-photon imaging, we used a similar confocal system connected to a MaiTai DeepSee Ti:sapphire laser with a tunable excitation range from 690–1,040 nm (Spectra Physics, Santa Clara, CA, USA). For measuring photostability of REX-GECO1 with two-photon excitation, HeLa cells expressing REX-GECO1 (treated with CaCl 2 (10 mM) and ionomycin (5 μM)) were imaged by two-photon microscopy with a × 20 XLUMPlanF1 water immersion objective (NA=1.00), and with excitation at 910 nm. Red fluorescent emission was acquired via a 605–680 nm bandpass filter (Semrock Inc, Rochester, NY, USA) with a frame resolution of 256 × 256 and a 10 μs per pixel scanning rate for 500 s. All images were processed and analyzed using ImageJ. Imaging of rat organotypic hippocampal slices The brain slice on the Millipore insert was placed in a custom-made chamber to hold it in place during imaging. Immediately before imaging, the slices were perfused with artificial cerebrospinal fluid (ACSF) containing: 120 mM NaCl, 3 mM KCl, 1 mM CaCl 2 , 2 mM MgSO 4 , 26 mM NaHCO 3 , 1.25 mM NaH 2 PO 4 and 10 mM D -glucose (pH adjusted to 7.4 by gassing with 95% O 2 , 5% CO 2 ), at 5 ml −1 min using a peristaltic pump (Watson-Marlow Alitea-AB, Sin-Can, Calgary, AB, Canada) and kept at room temperature. Imaging was started within 10 min following activation of the perfusion system. For single-colour one-photon imaging of REX-GECO1, the hippocampal slice was excited with 488 nm laser and emission was collected from 550 nm to 650 nm using a variable barrier filter. For single-colour one-photon imaging of Ca 2+ using R-GECO1 or RCaMP1h, the hippocampal slice was excited with 543 nm laser and emission was collected from 550 nm to 650 nm using a variable barrier filter. For dual-colour imaging of Ca 2+ using REX-GECO1 and glutamate using iGluSnFR, the slice was excited with 488 nm laser and emission was collected simultaneously in two channels from 500 to 520 nm for iGluSnFR and 590 to 690 nm for REX-GECO1 using variable barrier filters. In all cases, images were acquired at × 1–3 digital zoom at a reduced frame resolution (256 × 256) and with a 4 μs per pixel scanning rate. This allowed image acquisition to be 2–3 frame s- to detect Ca 2+ and glutamate oscillations in neurons ( Figs 3a,c and 4 ) and glial cells ( Fig. 3f,g ). For one-photon imaging of theophylline-induced Ca 2+ and/or glutamate rises in neurons, images were acquired every 0.5 s. Approximately 30 s after the start of the experiment, the superfusate was changed from control ACSF to ACSF containing 10 mM theophylline (Sigma-Aldrich, directly dissolved in ACSF). Approximately 10 min later, the superfusate was changed back to control ACSF. For KCl-evoked depolarization, 10 μl of (2.5 M) KCl was added to raise the concentration of KCl in the recording buffer to 30 mM instantaneously and then left to wash out at the regular rate of the perfusion system at 5 ml min −1 . For one-photon imaging of glutamate-induced Ca 2+ dynamics in glial cells, images were acquired every 0.5 s. Approximately 30 s after the start of the experiment, the superfusate was changed from control ACSF to ACSF containing 100 μM glutamate (Sigma-Aldrich, 1 M stock in dH 2 O, diluted to final concentration in control ACSF) for 10 min and then switched back to control ACSF. For two-colour two-photon imaging of REX-GECO1 and iGluSnFR, the laser wavelength was set at 940 nm. Fluorescence emission was collected using two photomultiplier tube detectors, one of which was equipped with a 460–500 nm bandpass filter, and the other equipped with a 605–680 nm bandpass filter (Semrock Inc, Rochester, NY, USA). Images were acquired every 0.25 s. Field potential recording LFP was recorded using a large-diameter patch pipette (outer tip diameter 5–15 μm, d.c. resistance 2–3 MΩ) micropipette pulled from borosilicate glass capillaries. The micropipette was filled with ACSF solution and placed ∼ 100 μm away from a REX-GECO1 transfected neuron. Electrode signals were amplified ( × 10 k) and bandpass filtered (0.3–1 kHz) (A-M systems, 1700, Carlsborg, WA, USA). Signals were then integrated ( τ : 15 ms) and digitally sampled at 1 kHz (Powerlab/8SP, ADInstruments, Colorado Springs, CO, USA), and stored on a computer using LabChart7 software (ADInstruments). REX-GECO1 fluorescence (imaged at 2 Hz) was imaged simultaneously using the same imaging setup described for imaging organotypic brain slices. Fluorescence images were processed and analyzed using ImageJ software. Electrical field stimulation of organotypic brain slices To stimulate hippocampal neurons in organotypic brain slices, a borosilicate glass capillary electrode (outer tip diameter 30–40 μm) attached to an ISO-Flex pulse stimulator (A.M.P.I.) was placed ∼ 500 μm away from the transfected neurons. The electrode was manoeuvered using a ROE-200 micromanipulator (Sutter Instruments, Novato, CA, USA). Field stimulation pulses (4 V, 1 ms, 100 Hz) were delivered in trains of 1, 3, 5, 10, 20, 50 and 150 pulses using Powerlab/8SP (ADInstruments) to control the pulse stimulator. Each field stimulation pattern was repeated twice. Fluorescence signals (imaged at 2 Hz) induced by field electrode stimulation was recorded using the same imaging setup described for imaging organotypic brain slices. Fluorescence images were processed and analyzed using ImageJ software. In vivo experimental animals Albino X. laevis tadpoles were bred by human chorionic gonadotropin-induced mating. Embryos were reared at room temperature in 0.1 × modified Barth’s saline with HEPES (MBSH). Tadpoles were developmentally staged according to the standard criteria of Nieuwkoop and Faber [48] . Experiments were approved by the Montreal Neurological Institute Animal Care Committee in accordance with Canadian Council on Animal Care guidelines. In vivo electroporation Cells in the retina and optic tectum were bulk electroporated as described previously [49] . In brief, glass micropipettes made from borosilicate capillaries pulled on a PC-10 puller (Narishige, Japan) were loaded with DNA plasmid solution (0.5–5 μg μl −1 ) and attached to a custom-made pressure injection system. Plasmid solution was then pressure-injected in the eye or brain ventricle and current was locally delivered across custom-made platinum plate electrodes placed on either side of the eye, or the tectum using three pulses (36 V, 1.6 ms) in each polarity using a constant voltage stimulator (Grass SD-9) with a 3 μF capacitor placed in parallel. In vivo imaging of Xenopus tadpoles Stage 40 tadpoles for retinal electroporation and stage 43 for tectal electroporation were transfected with plasmids encoding REX-GECO1 mixed with EGFP-encoding plasmid, and given at least 48 h to express the protein. Stage 45–47 tadpoles were immobilized by bath application of pancuronium bromide (2 mM, Sigma) and placed in a custom-made imaging chamber, embedded in 1% low-melting point agarose, and then immersed in modified Barth s saline with HEPES (MBSH) solution for tectal cell imaging and with ACSF external solution for retinal imaging. The ACSF solution contains 115 mM NaCl, 2 mM KCl, 5 mM HEPES, 3 mM CaCl 2 , 1.5 mM MgCl 2 , 10 mM D -glucose, 5 μM glycine; 250 mOsm; pH 7.2. In vivo two-photon images of tectal cells or retinal cells were acquired at 2 and 5 Hz, respectively, using a Thorlabs multiphoton microscope with resonant scanner and Olympus × 20 1.0 NA immersion objective, A MaiTai-BB Ti:sapphire femtosecond pulsed laser set to excite at 910 nm was used for fluorescence excitation. Green (500–550 nm) and red (584–676 nm) emission filters were used for fluorescence detection. For visual stimulation, an A310 Accupulser (WPI) was used to drive a blue LED (447.5 nm, royal-blue Luxeon Star) to present trains of light flashes. Ex vivo imaging of tadpole brains Stage 45–47 tadpoles were anesthetised by immersion in 0.02% MS-222 and the brain was dissected and perfused with Mg-free external solution containing 115 mM NaCl, 2 mM KCl, 5 mM HEPES, 3 mM CaCl 2 , 10 mM D -glucose, 10 μM glycine; 250 mOsm; pH 7.2. Imaging was carried out at 910 nm using an Olympus FV300 confocal microscope converted for multiphoton use, with a × 40 1.0 NA immersion objective. For pharmacological activation of N-methyl-D-aspartate receptors (NMDARs), 20 μM NMDA was applied to the bath. To visualize fluorescence intensity changes, images of the tectum were acquired at 2 Hz simultaneously on green (500–550 nm) and red (593–668 nm) channels. At the end of each experiment, z-series stacks at 1 μm inteval were collected to obtain full three-dimensional cellular morphologies. Fluorescence intensity change analysis Ellipsoid ROIs were selected manually around visually identifiable somata, or complex ROIs were drawn around axons or dendrites and the mean intensity of the ROIs in both the green and the red channel was determined for each frame from the time series using ImageJ (NIH). The background intensity was measured by calculating the mean intensity of a large ROI in an area without any fluorescent structures. For each frame, the background intensity was subtracted from the intensity of the ROI of the cell compartment of interest. For the in vivo visual stimulation, F 0 was calculated as an average of the (ROI intensity−background intensity) for the initial 25 frames baseline period before the beginning of the light flashes. The change in fluorescence was measured as Δ F / F 0 , where Δ F = F (t) − F 0 . For the ex vivo pharmacological preparation for each time point the following ratio ( R ) was calculated: . R 0 was calculated as an average of R during the initial 37 s baseline before application of drug. The change of fluorescence intensity was measured as Δ R / R 0 , where Δ R = R (t) – R 0 . Statistics Two-tailed Student’s t -tests were used to determine significance. How to cite this article: Wu, J. et al. A long Stokes shift red fluorescent Ca 2+ indicator protein for two-photon and ratiometric imaging. Nat. Commun. 5:5262 doi: 10.1038/ncomms6262 (2014).